The emerging biofuel cropCamelina sativaretains a highly undifferentiated hexaploid genome structure Camelina sativa is an oilseed with desirable agronomic and oil-quality attributes for a viable industrial oil platform crop. Here we generate the first chromosome-scale high-quality reference genome sequence for C. sativa and annotated 89,418 protein-coding genes, representing a whole-genome triplication event relative to the crucifer model Arabidopsis thaliana . C. sativa represents the first crop species to be sequenced from lineage I of the Brassicaceae. The well-preserved hexaploid genome structure of C. sativa surprisingly mirrors those of economically important amphidiploid Brassica crop species from lineage II as well as wheat and cotton. The three genomes of C. sativa show no evidence of fractionation bias and limited expression-level bias, both characteristics commonly associated with polyploid evolution. The highly undifferentiated polyploid genome of C. sativa presents significant consequences for breeding and genetic manipulation of this industrial oil crop. C amelina sativa (false flax or gold of pleasure) is a relict oilseed crop of the Crucifer family (Brassicaceae) with centres of origin in southeastern Europe and southwestern Asia. C. sativa was cultivated in Europe as an important oilseed crop for many centuries before being displaced by higher-yielding crops such as canola ( Brassica napus ) and wheat. C. sativa has several agronomic advantages for production, including early maturity, low requirement for water and nutrients, adaptability to adverse environmental conditions and resistance to common cruciferous pests and pathogens [1] , [2] , [3] . With seed oil content (36–47%) [2] twice that of soybean (18–22%) [2] and a fatty acid profile (with >90% unsaturated fatty acids) suitable for making jet fuel, biodiesel and high-value industrial lubricants, C. sativa has tremendous potential to serve as a viable and renewable feedstock for multiple industries. Additionally, due to exceptionally high levels of α-linolenic acid (32–40% of total oil content) [2] , C. sativa oil offers an additional source of essential fatty acids. The residual essential fatty acids combined with low glucosinolate levels in C. sativa meal make it desirable as an animal feed. Considering the broad applications, C. sativa is currently being re-embraced as an industrial oil platform crop; however, due to limited availability of genetic and genomic resources, the full agronomic and breeding potential of this emerging oilseed crop remains largely unexploited. Genetically, C. sativa is closely related to the model plant Arabidopsis thaliana (lineage I of the Brassicaceae) and more distantly to the important vegetable oilseed crop, canola (lineage II) [4] . The previously estimated genome size (750 Mb) [5] and chromosome count ( n =20) of C. sativa are higher compared with most of the Brassicaceae species that have been sequenced to date ( Supplementary Fig. 1 ). However, the genetic basis for the genome expansion of C. sativa is currently unknown. In many plant taxa, polyploidization and proliferation of transposable elements (TEs) are recognized as prevalent factors in plant genome expansion [6] , [7] . Similar to the diploid progenitors of canola ( B. rapa and B. oleracea ) [8] , [9] , C. sativa is suggested to have undergone a genome triplication event [5] . However, the evolutionary origin and mode of the polyploidization event that formed the C. sativa genome as well as the post-polyploidization evolutionary path leading to its diploidization are currently not understood. Here we sequence a homozygous doubled haploid line of C. sativa and assembled 82% of the estimated genome size in order to decipher the genome organization of C. sativa and facilitate development of genetic and genomic tools essential for crop improvement. The genome sequence of C. sativa will provide an indispensable tool for genetic manipulation and further crop improvement. Genome sequencing and assembly The genome of a homozygous doubled haploid line of C. sativa (DH55) was sequenced using a hybrid Illumina and Roche 454 next-generation sequencing (NGS) approach ( Supplementary Note 1 ; Supplementary Fig. 2 ). 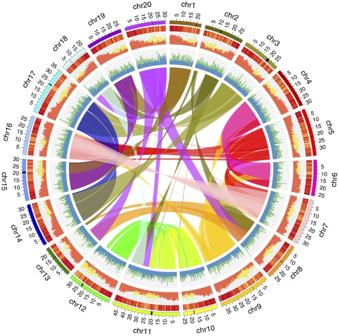Figure 1: TheCamelina sativagenome. From the outside ring to the centre: (1) the twentyC. sativapseudochromosomes (Chr1–20 represented on Mb scale) are shown in different colours with putative centromeric regions indicated by black bands; (2) gene expression levels (log10(average FPKM), bin=250 Kb)), values range from 0 (yellow) to 3.92 (red); (3) the distribution of protein-coding regions (nucleotides per 500 Kb; orange) compared with repetitive sequences (nucleotides per 500 Kb; yellow); and (4)Ka/Ksratios (median, bin=500 kb) of syntenic (blue) and non-syntenic (green) genes. The centre shows a graphical view of the triplicated segments of annotated genes connected with lines of colours matching those for the pseudochromosomes. Filtered sequence data (96.53 Gb) provided 123 × coverage ( Supplementary Table 1 ) of the estimated genome size of 785 Mb ( Supplementary Note 2 ; Supplementary Fig. 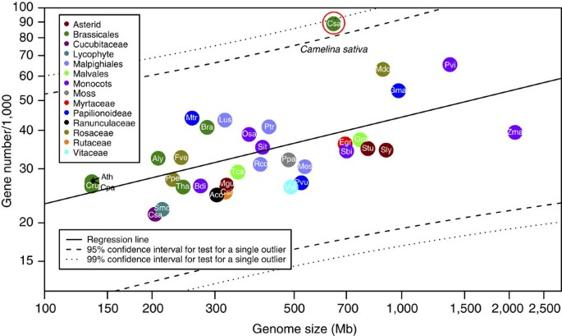Figure 2: Comparison of gene number inC. sativaplotted against genome size with a subset of completely sequenced plant genomes (N=35). The significance test for a single outlier in regression data was performed as described in detail inSupplementary Note 8and the confidence intervals for the regression line are shown as dotted lines. Mes,Manihot esculenta; Rco,Ricinus communis; Lus,Linum usitatissimum; Ptr,Populus trichocarpa; Mtr,Medicago truncatula; Pvu,Phaseolus vulgaris; Gma,Glycine max; Csa,Cucumis sativis; Ppe,Prunus persica; Mdo,Malus domestica; Fve,Fragaria vesca; Ath,Arabidopsis thaliana; Aly,Arabidopsis lyrata; Csa,Camelina sativa; Cru,Capsella rubella; Bra,Brassica rapa; Tha,Thellungiella halophila; Cpa,Carica papaya; Gra,Gossypium raimondii; Tca,Theobroma cacao; Csi,Citrus sinensis; Egr,Eucalyptus grandis; Vvi,Vitis vinifera; Stu,Solanum tuberosum; Sly,Solanum lycopersicum; Mgu,Mimulus guttatus; Aco,Aquilegia coerulea; Sbi,Sorghum bicolour; Zma,Zea mays; Sit,Setaria italica; Pvi,Panicum virgatum; Osa,Oryza sativa; Bdi,Brachypodium distachyon; Smo,Selaginella moellendorfii; Ppa,Physcomitrella patens. 3 ), which was assembled using a hierarchical assembly strategy ( Supplementary Note 1 ) into 37,871 scaffolds, with a sequence span of 641.45 Mb and an N50 size of 2.16 Mb ( Supplementary Table 2 ). A high-density genetic map based on 3,575 polymorphic markers allowed 608.54 Mb of the assembled genome, represented by 588 scaffolds to be anchored to the 20 chromosomes of C. sativa ( Fig. 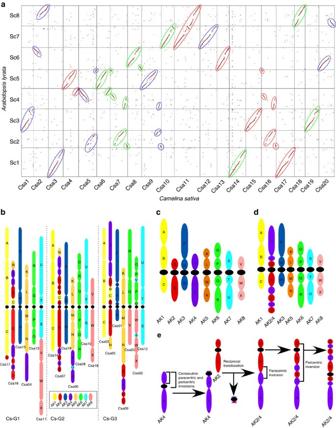Figure 3: Comparative analysis and evolution of theC. sativagenome. (a) MUMer plot comparing theC. sativaandA. lyratagenomes. Syntenic and collinear regions making the three complete sub-genomes inC. sativaare circled in red, blue and green. (b) Reconstruction of the three sub-genomes ofC. sativa.Chromosome and ancestral genomic-block-level organization of the sub-genomes inC. sativais shown. Based on synteny and collinearity betweenC. sativaandArabidopsisspecies, and GB contiguity in the ancestral karyotype, pseudochromosomes were assigned to three sub-genomes inC. sativa. Each pseudochromosome was subdivided among ancestral genomic blocks (A–X), which are coloured based on their occurrence in the ACK. (c) ACK consisting of the 24 conserved genomic blocks (A–X). (d) The ancestral diploid karyotype (derivative of ACK) ofC. sativa. (e) The presumed origin and reconstruction of the fusion chromosome (AK2/4) of the dACK. 1 ; Supplementary Table 3 ), thereby producing a highly contiguous final assembly with an N50 size of >30 Mb ( Supplementary Table 2 ). The final genome assembly contains 641.45 Mb of sequence, covering 82% of the estimated genome size, 95% of which is in 20 chromosomes. 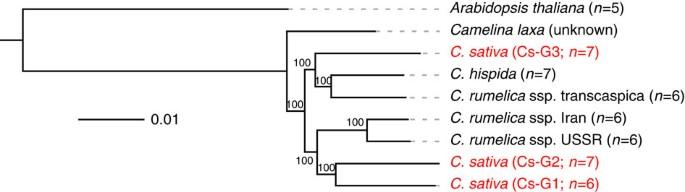Figure 4: Phylogenetic relationship between the three sub-genomes ofC. sativaand lower-chromosomeCamelinaspecies. A maximum-likelihood tree produced from a supermatrix constructed using 4,867 orthologous sequences. Clade support values near nodes represent bootstrap proportions in percentages. Branch lengths represent estimated nucleotide substitutions per site. A summary describing the overall features as well as completeness and contiguity of the genome assembly is provided in Supplementary Table 4 . Comparison of the genome sequence with a set of independently assembled BAC scaffolds, expressed sequence tags (ESTs) and core eukaryotic genes ( Supplementary Note 3 ; Supplementary Tables 5–8 ) confirmed the quality as well as near complete coverage of the euchromatic space and gene complement in the assembly. Figure 1: The Camelina sativa genome. From the outside ring to the centre: (1) the twenty C. sativa pseudochromosomes (Chr1–20 represented on Mb scale) are shown in different colours with putative centromeric regions indicated by black bands; (2) gene expression levels (log10(average FPKM), bin=250 Kb)), values range from 0 (yellow) to 3.92 (red); (3) the distribution of protein-coding regions (nucleotides per 500 Kb; orange) compared with repetitive sequences (nucleotides per 500 Kb; yellow); and (4) Ka / Ks ratios (median, bin=500 kb) of syntenic (blue) and non-syntenic (green) genes. The centre shows a graphical view of the triplicated segments of annotated genes connected with lines of colours matching those for the pseudochromosomes. Full size image Repeat annotation and gene prediction Repeat annotation revealed that 28% (180.12 Mb) of the assembled C. sativa genome comprises TEs ( Supplementary Table 9 ). Retrotransposons were found to be the dominant class of repeat elements (19%), while DNA transposons accounted for 3% of the genome. Similar to most higher plant genomes, repetitive elements in C. sativa were more abundant in the vicinity of centromeres and less so in gene-dense regions ( Fig. 1 ). The genome occupancy of repetitive DNA in C. sativa (28%) is comparable to the low abundance of TEs in A. thaliana (24%) [10] and A. lyrata (30%) [10] . However, it is much smaller than in B. rapa (39.5%) [7] as well as other similar-sized plant genomes, including potato (62%) [11] , soybean (59%) [12] and sorghum (62%) [13] . Thus, unlike B. rapa and other angiosperm species, genome expansion in C. sativa has not resulted from repetitive sequence proliferation. RNA-seq data (78.5 Gb) was generated from tissue samples collected at 12 different growth stages to assist with annotation of protein-coding genes ( Supplementary Table 10 ). Based on a comprehensive strategy of ab initio gene prediction and homology evidence from proteome data sets, ESTs and RNA-seq transcripts ( Supplementary Fig. 4 ), 89,418 non-redundant C. sativa genes were predicted, of which 4,753 (5.3%) genes encoded two or more alternatively spliced isoforms ( Supplementary Table 4 ). More than 95% (85,274) of these annotated genes were located on the pseudochromosomes with the remainder on unanchored scaffolds. The overall gene model characteristics, such as gene length and exon-intron structures are comparable to other Brassicaceae species ( Supplementary Fig. 5 ). The genome composition (genic, intergenic and repeat regions) of C. sativa is more similar to that of A. lyrata [10] than A. thaliana ( Supplementary Table 11 ). Based on sequence identity a total of 86,849 (97.13%) of the predicted C. sativa genes have homologues in the UniProt database ( Supplementary Data 1 ), and RNA-seq evidence suggested that >90% of the genes were expressed (FPKM>0) in one or more developmental stages ( Fig. 1 ). The genome sequence and its annotation are available along with a genome browser at http://www.camelinadb.ca . The predicted number of protein-coding genes in C. sativa is significantly higher than other currently sequenced plant genomes ( Fig. 2 , Supplementary Table 12 ). Interestingly, the gene number is similar to that predicted for bread wheat whose genome is almost 22 times larger than that of C. sativa [14] . The estimated total number of genes in C. sativa is approximately three times that of the model Arabidopsis species ( Supplementary Table 11 ), suggesting that the C. sativa genome resulted from a whole-genome triplication of a common ancestor. To determine whether the expanded gene repertoire in C. sativa could have arisen from an expansion of lineage-specific C. sativa orphan genes [15] , we used a BLAST-based filtering approach comparing C. sativa genes with all sequenced plant taxa excluding the five Brassicaceae species. A total of 3,761 Brassicaceae-specific orphan genes were identified, of which 1,656 were C. sativa –specific, which accounts for only 1.85% of annotated protein-coding genes in C. sativa ( Supplementary Note 4 ; Supplementary Tables 13 and 14 ). Figure 2: Comparison of gene number in C. sativa plotted against genome size with a subset of completely sequenced plant genomes ( N =35). The significance test for a single outlier in regression data was performed as described in detail in Supplementary Note 8 and the confidence intervals for the regression line are shown as dotted lines. Mes, Manihot esculenta ; Rco, Ricinus communis ; Lus, Linum usitatissimum ; Ptr, Populus trichocarpa ; Mtr, Medicago truncatula ; Pvu, Phaseolus vulgaris ; Gma, Glycine max ; Csa, Cucumis sativis ; Ppe, Prunus persica ; Mdo, Malus domestica ; Fve, Fragaria vesca ; Ath, Arabidopsis thaliana ; Aly, Arabidopsis lyrata ; Csa, Camelina sativa ; Cru, Capsella rubella ; Bra, Brassica rapa ; Tha, Thellungiella halophila ; Cpa, Carica papaya ; Gra, Gossypium raimondii ; Tca, Theobroma cacao ; Csi, Citrus sinensis ; Egr, Eucalyptus grandis ; Vvi, Vitis vinifera ; Stu, Solanum tuberosum ; Sly, Solanum lycopersicum ; Mgu, Mimulus guttatus ; Aco, Aquilegia coerulea ; Sbi, Sorghum bicolour ; Zma, Zea mays ; Sit, Setaria italica ; Pvi, Panicum virgatum ; Osa, Oryza sativa ; Bdi, Brachypodium distachyon ; Smo, Selaginella moellendorfii ; Ppa, Physcomitrella patens . Full size image Synteny and collinearity with Brassicaceae species The genome sequence and gene annotations of C. sativa were compared with those of phylogenetically closely related Brassicaceae species ( Supplementary Fig. 6 ), including A. thaliana (model Crucifer species), A. lyrata (reference for ancestral karyotype) and B. rapa (reference for polyploidization). Chromosomal collinearity assessed through whole-genome alignments revealed a striking level of conservation between the genome sequence of C. sativa and the two Arabidopsis species ( Fig. 3a ; Supplementary Fig. 7 ). The longest stretches of conserved syntenic blocks were observed between the C. sativa and A. lyrata genomes ( Fig. 3a ), with syntenic regions spanning almost complete chromosomes from both of these species. Notably, every chromosome or chromosomal region in A. lyrata or A. thaliana was represented in three independent chromosomes in the C. sativa genome, thus providing robust evidence for a whole-genome triplication event. Figure 3: Comparative analysis and evolution of the C. sativa genome. ( a ) MUMer plot comparing the C. sativa and A. lyrata genomes. Syntenic and collinear regions making the three complete sub-genomes in C. sativa are circled in red, blue and green. ( b ) Reconstruction of the three sub-genomes of C. sativa. Chromosome and ancestral genomic-block-level organization of the sub-genomes in C. sativa is shown. Based on synteny and collinearity between C. sativa and Arabidopsis species, and GB contiguity in the ancestral karyotype, pseudochromosomes were assigned to three sub-genomes in C. sativa . Each pseudochromosome was subdivided among ancestral genomic blocks (A–X), which are coloured based on their occurrence in the ACK. ( c ) ACK consisting of the 24 conserved genomic blocks (A–X). ( d ) The ancestral diploid karyotype (derivative of ACK) of C. sativa . ( e ) The presumed origin and reconstruction of the fusion chromosome (AK2/4) of the dACK. Full size image Reconstructing the three sub-genomes of hexaploid C. sativa The triplicated chromosomal segments in C. sativa were identified and assigned to a sub-genome using the protein-coding genes from A. thaliana as discrete genomic anchors to determine the corresponding syntenic orthologues (syntelogs) from C. sativa and the extent of the collinear conserved block environment. A syntelog matrix representing individual A. thaliana genes and the corresponding triplets of C. sativa homologues is presented in Supplementary Data 2 . A total of 62,277 C. sativa genes were found to be syntenically orthologous to A. thaliana genes; these genes will be referred to as ‘syntelogs’, and the remaining 27,141 genes are divided into tandem duplicates (10,792 genes) and ‘non-syntenic genes’ (16,349 genes). Syntelogs were further classified as either ‘fully retained’ (if all three homologues were retained) or ‘fractionated’ (if one or two of the homologues were lost). Comparative mapping and cytogenetic studies have suggested that most of the Brassicaceae species have evolved from an ancestral karyotype comprising 8 chromosomes and 24 conserved genomic blocks (labelled as A–X) [16] . To decipher the nature of the ancestral karyotype of C. sativa , its genomic block (GB) structure was elucidated based on previously defined GB intervals in A. thaliana [17] . As expected, for each A. thaliana GB three syntenic copies were detected in C. sativa ( Supplementary Fig. 8 ). Of the 24 GBs, 20 were found to be maintained in three nearly undisrupted copies, whereas the remaining four GBs (D, E, I and J) exhibited rearrangements ( Supplementary Fig. 8 ). Utilizing the extensive synteny and collinearity between C. sativa and Arabidopsis species, GB contiguity in the ancestral karyotype, and the assumption that syntenic fragments of each C. sativa chromosome derive from the same ancestral chromosome, the most parsimonious path to sub-genome structure was deduced (discussed in Methods) and the triplicated sub-genomes within C. sativa were reconstructed ( Fig. 3b ). Accordingly, sub-genome I of C. sativa (Cs-G1) contains six chromosomes, while the other two sub-genomes (Cs-G2 and Cs-G3) contain seven chromosomes each ( Fig. 3b ). The sub-genomes each encode 28,274, 27,218 and 29,207 genes, respectively ( Supplementary Table 15 ), which are highly comparable to the A. thaliana gene complement. Deciphering the ancestral karyotype of C. sativa The organization of the GBs in C. sativa was compared with previously inferred ancestral karyotypes, including the ancestral crucifer karyotype (ACK; n =8) [16] , proto-calepineae karyotype (PCK; n =7) [18] and translocated PCK (tPCK [17] ; n =7; Supplementary Table 16 ). All 16 GB associations that were defined in ACK were conserved in C. sativa but only 11 of 17 GB associations defined for PCK and tPCK were identified ( Supplementary Table 16 ), suggesting that C. sativa genome organization is more similar to the ACK ( Fig. 3c ). However, a number of additional unique GB associations observed in C. sativa , such as D/I, E/I, N/J, Q/V, O/W and O/R have not been reported in ancestral Brassicaceae karyotypes defined so far. Only two of these novel GB associations D/I and E/I were common to all three sub-genomes within C. sativa ( Fig. 3b ). Additionally, Csa16, Csa7 and Csa5/9 from Cs-G1, Cs-G2 and Cs-G3, respectively, carrying these two novel GB associations display further rearrangements resulting in a common organization of GBs as J/I/D/E/I/E/I/D ( Fig. 3b ), suggesting the pre-existence of this novel GB structure in the parental karyotype from which the three sub-genomes of C. sativa evolved. Based on the above observations, the putative diploid karyotype of C. sativa , named dACK (derivative of ACK), comprising seven chromosomes ( Fig. 3d ) was inferred. The dACK karyotype ( n =7) comprises six ancestral chromosomes (AK1, 3, 5, 6, 7 and 8) and a chromosomal fusion (AK2/4) ( Fig. 3e ; Supplementary Fig. 9 ; Supplementary Data 2 ). Previous karyotype analyses of C. sativa and related Camelina species has detailed a range of chromosome numbers including n =6, 7, 13 and 20 (ref. 19 ). The lower chromosome numbers are consistent with the dACK karyotype and the identified sub-genomes. The higher chromosome counts could suggest that two independent hybridization events resulted in the current hexaploid genome. However, without reference to extant diploid relatives of each sub-genome it is difficult to accurately determine the origin of C. sativa . EST contigs derived from 454 pyrosequencing of the leaf transcriptome of five representatives of all known lower chromosome number Camelina species were used to derive the phylogenetic relationship between these species and the three sub-genomes ( Fig. 4 ; Supplementary Note 5 ). The genomes of Cs-G1 and Cs-G2 are more closely related to each other than any of the diploids assayed, which could suggest an initial tetraploidisation event of two closely related species (that is, possibly an amphidiploid), subsequently followed by an additional hybridization event through which Cs-G3 joined, resulting in a hexaploid genome. Figure 4: Phylogenetic relationship between the three sub-genomes of C. sativa and lower-chromosome Camelina species. A maximum-likelihood tree produced from a supermatrix constructed using 4,867 orthologous sequences. Clade support values near nodes represent bootstrap proportions in percentages. Branch lengths represent estimated nucleotide substitutions per site. Full size image Analysis of the distribution of synonymous substitutions ( K s) among the coding regions of paralogous gene pairs provided an estimate of the age of divergence of the three sub-genomes in C. sativa . Mixture model analysis of the K s distribution uncovered the previously documented Brassicaceae-related α, β and γ paleopolyploidy events, and revealed the presence of an additional peak at K s=~0.09 ( Fig. 5 ; Supplementary Fig. 10 ). Assuming an established synonymous substitution rate of 8.22 × 10 −9 substitutions/synonymous site/year for Brassicaceae species [20] , the three genomes of C. sativa were estimated to have separated ~5.41 million years ago (Mya), which is comparable to the divergence time of the three mesopolyploid (functionally diploid) Brassica genomes ( B. oleracea , B. rapa and B. nigra ) that fused in all pairwise combinations to form the allopolyploid crop species B. napus (canola), B. juncea (oriental mustard) and B. carinata (Ethiopian mustard) [21] . The mesopolyploid structure of the Brassica diploid genomes exhibit extensive reduction of chromosome number and rearrangement of ancestral chromosomal blocks. This structure is also mirrored in Australian Brassicaceae species, including Stenopetalum and Ballantinia species that diverged ~5.9 Mya (ref. 22 ). The relatively unarranged nature of the C. sativa sub-genomes with respect to A. thaliana and A. lyrata stands in contrast to these observations but could reflect a more highly conserved nature of these species within the Camelineae tribe. The three sub-genomes within C. sativa , although showing some differentiation at the nucleotide-level (2–2.5% sequence variation across the coding regions), share a similar gene complement. The hybridization of sub-genomes in C. sativa probably occurred relatively recently, similar to the Brassica crop allopolyploids, resulting in insufficient time for the differentiation of gene complement within the three sub-genomes. Comparisons of pairs of syntelogs found between the three sub-genomes and A. thaliana revealed almost identical K s distributions with a major peak at 0.28 ( Fig. 5 ), suggesting that the diploid parents of the triplicated C. sativa sub-genomes shared a common ancestor that diverged from A. thaliana ~17 Mya. 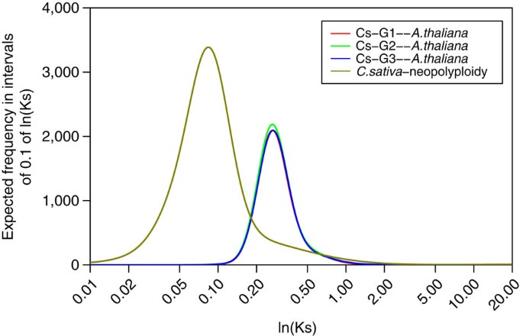Figure 5: Age distribution of duplicated genes inC. sativa. Gaussian mixture models fitted to frequency distributions ofKs (synonymous substitution) values obtained by comparing pairs of paralogous (C. sativa—neopolyploidy) and orthologous (Sub-genomes 1/2/3versus A. thaliana) genes are shown. The mixture model analysis is described inSupplementary Note 9and the complete list of Gaussian components is provided inSupplementary Table 23. Figure 5: Age distribution of duplicated genes in C. sativa . Gaussian mixture models fitted to frequency distributions of K s (synonymous substitution) values obtained by comparing pairs of paralogous ( C. sativa —neopolyploidy) and orthologous (Sub-genomes 1/2/3 versus A. thaliana ) genes are shown. The mixture model analysis is described in Supplementary Note 9 and the complete list of Gaussian components is provided in Supplementary Table 23 . Full size image Homeologous gene expression bias and genome dominance After polyploidization, duplicated genomes enter an evolutionary trajectory of genetic diploidization during which the nearly identical sub-genomes differentiate via biased loss of homologous genes (fractionation), which is commonly associated with overexpression of genes from the least fractionated sub-genome (genome dominance) [7] , [23] , [24] , [25] , [26] , [27] , [28] . Preceding genome fractionation is a period of ‘genomic shock’ when a mixture of genetic and epigenetic mechanisms is proposed to lead to neo- or subfunctionalization of duplicated genes. Enumeration of syntelogs revealed that the three sub-genomes (Cs-G1, Cs-G2 and Cs-G3) of C. sativa have retained an almost identical number of genes ( Supplementary Table 17 ), which compares starkly with the differentially fractionated LF, MF1 and MF2 sub-genomes of B. rapa that have retained only 13,296, 8,891 and 7,659 genes, respectively ( Supplementary Fig. 11 ). However, it is noteworthy that the rate of gene loss in all three sub-genomes of C. sativa (5% of genes per million year (Myr) is identical to the rate of gene loss in the MF1 sub-genome of B. rapa (5% of genes per Myr; Supplementary Table 18 ), indicating that the sub-genomes of C. sativa despite lacking a fractionation bias are experiencing the expected exponential decay pattern of gene loss immediately following whole-genome duplication [29] . Deletion of exonic sequences is one of the mechanisms by which genes are potentially rendered non-functional and subsequently removed from polyploid genomes [26] . Comparing the coding sequences of homeologous genes within triplicated regions demonstrated that both the number of exons and length of coding sequences in syntelogs were highly conserved ( Supplementary Table 19 ), indicating that limited insertions or deletions have accumulated in coding sequences of C. sativa within the last 5.5 Myrs. Gene expression levels are a major determinant of the fate of duplicated copies following whole-genome duplication. It has been shown that the rate of gene loss post polyploidisation may be negatively correlated to the level of gene expression [30] . Comparison of the expression levels of fully retained and fractionated sets of C. sativa genes revealed a positive correlation between retention rate of triplicated homeologues and their average expression levels ( Fig. 6a ), suggesting that highly expressed genes tend to persist longer. Evidence of genome dominance in C. sativa was assessed by comparing expression differences between the sub-genomes of C. sativa based on transcript abundance of genes across 12 different tissue types (listed in Supplementary Table 10 ). Only the fully retained homeologues were included in this analysis to avoid discrepancy due to fractionation. At sub-genome (G) and tissue-type (T) interaction (G × T) level a statistically significant difference was revealed ( P <0.05; ANOVA test for interaction) for 77% (14,391 triplets) of fully retained homeologues. The genes of sub-genome Cs-G3 showed a clear expression level advantage over the other two sub-genomes ( Fig. 6b ), which could result from a two-stage polyploidisation pathway. 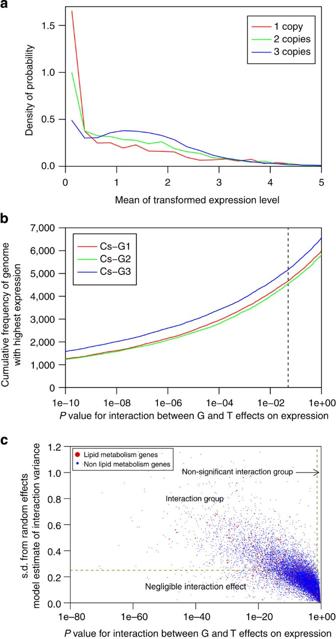Figure 6: Gene expression dynamics reveal genome dominance and functional diversification ofC. sativahomeologous genes. (a) Relationship between gene retention rate following whole-genome triplication and the gene expression levels. (b) Cumulative frequency of homeologous genes belonging to the three sub-genomes withinC. sativawith highest expression across all tissue types.Pvalues (ANOVA test for interaction,N=108 per gene triplet) were calculated for interaction between sub-genomes (G) and tissue-type (T) effects on expression. To highlight differences between sub-genomes only the subset of the data withP>10−10is shown. (c) Scatterplot showing the magnitude of interaction effect calculated as the s.d. from a random effects model estimate for G × T interaction variance. Homeologous triplets were classified into groups, no interaction (P>0.05; ANOVA test for interaction,N=108), negligible interaction (P<0.05 and STDEV(G × T)<0.25) and interaction (P<0.05 and STDEV(G × T)>0.25). Figure 6: Gene expression dynamics reveal genome dominance and functional diversification of C. sativa homeologous genes. ( a ) Relationship between gene retention rate following whole-genome triplication and the gene expression levels. ( b ) Cumulative frequency of homeologous genes belonging to the three sub-genomes within C. sativa with highest expression across all tissue types. P values (ANOVA test for interaction, N =108 per gene triplet) were calculated for interaction between sub-genomes (G) and tissue-type (T) effects on expression. To highlight differences between sub-genomes only the subset of the data with P >10 −10 is shown. ( c ) Scatterplot showing the magnitude of interaction effect calculated as the s.d. from a random effects model estimate for G × T interaction variance. Homeologous triplets were classified into groups, no interaction ( P >0.05; ANOVA test for interaction, N =108), negligible interaction ( P <0.05 and STDEV(G × T)<0.25) and interaction ( P <0.05 and STDEV(G × T)>0.25). Full size image Only 4,106 of the 14,391 triplets revealed an interaction effect of considerable magnitude (STDEV (G × T) >0.25; Fig. 6c ; Table 1 ); this set was designated as the ‘interaction group’ ( Fig. 6c ). Since the differential expression profiles may result from divergent fates of the triplicated genes, further analyses determined the levels of non-functionalization (silencing), neofunctionalization (diversification) or subfunctionalization (shared and/or partitioned functions). Across all 12 tissue types, ~5% of the fully retained homeologues were found to be silenced (FPKM=0 in one or two sub-genomes) ( Table 1 ; Supplementary Table 20 ) with the non-expressed homeologues being equally distributed across all three sub-genomes. Hierarchical clustering of all 12,212 genes belonging to the interaction group based on patterns of gene expression across all 12 tissue types revealed seven major clusters ( Supplementary Fig. 12 ). Genes belonging to each cluster were predominantly expressed in one or a few tissue types, suggesting potential tissue-specific functions. However, genes from 34% (1,316) of the homeologous triplets clustered together; with the remaining 66% being separated across two (699 triplets) or three (1,904 triplets) independent clusters. As homeologues with altered expression patterns potentially may acquire new or additional functions, the results provide evidence for functional diversification of a subset of triplicated genes within C. sativa . The majority of the triplicated genes (78%) showed no significant differences in either expression levels or tissue specificity, which could impact manipulation of the crop phenotype. Table 1 Incidence of expression and functional diversification of fully retained acyl-lipid metabolism related genes in C. sativa . Full size table Oil metabolism genes In the context of the importance of C. sativa as a biofuel crop, we examined the fractionation and expression divergence of genes encoding proteins and regulatory factors involved in acyl-lipid metabolism [31] . More than 80% of the 736 non-redundant genes [31] governing various steps in acyl-lipid biosynthesis, accumulation and degradation were found to be retained in three copies ( Supplementary Table 21 ). A subset of the acyl-lipid metabolism genes (26%), mainly involved in fatty acid and triacylglycerol biosynthesis, elongation or degradation, experienced further expansion with a few genes, such as CER1 and WS (both involved in fatty acid elongation and wax biosynthesis) and LOX (involved in oxylipin metabolism), having >10 paralogues ( Supplementary Data 3 ). The overall expansion of lipid metabolism gene families in C. sativa (217% compared with A. thaliana ) is significantly larger than in soybean (63% increase compared with A. thaliana ) [12] . Analysis of expression divergence revealed significant differences among only 31% (181 triplets) of the fully retained lipid metabolism genes ( Fig. 6c ; Table 1 ). Hierarchical clustering of genes belonging to this set revealed that only 15% of acyl-lipid metabolism genes were experiencing functional diversification ( Table 1 ). The higher retention of lipid metabolism genes in C. sativa does not necessarily reflect adaptation of an oilseed phenotype and could merely be a consequence of polyploidy; however, the larger number of genes involved in lipid metabolism in C. sativa , with the majority showing no expression or functional divergence, suggests that complex regulatory mechanisms govern oil biosynthesis to ensure gene dosage balance. The knowledge of copy number, genomic context and regulation of oil metabolism genes will aid in the future manipulation of biofuel traits in C. sativa. C. sativa is an excellent model that exemplifies the selection of a crop ecotype from a weedy ancestor. Without knowledge of the parental diploids it is difficult to predict the exact origin of C. sativa ; however, the strict maintenance of homologous recombination between highly syntenic sub-genomes suggests that like many successful crop species C. sativa may have been formed through inter-specific hybridization of lower chromosome number ancestors. The emerging signatures of genome dominance and functional diversification among a subset of genes in C. sativa are largely concordant with the characteristics of genomic shock triggered by hybridization and dosage imbalance during allopolyploid formation [29] . The genome sequence strongly supports the hypothesis that the relatively large genome size and high gene content of C. sativa are the consequence of two polyploidy events from an ancestral genome similar to A. lyrata . The minimal chromosomal rearrangements and lack of widespread or biased fractionation in the three C. sativa sub-genomes suggests that the hybridization of the sub-genomes occurred in quick succession and relatively recently, probably emerging on the same time scale as crops such as canola, cotton or wheat, during the rapid expansion of agricultural practices 5–10,000 ya. It is remarkable that despite having nearly identical sub-genomes C. sativa behaves like a diploid with normal disomic inheritance. The age of divergence of the three genomes (5 Mya) may have been sufficient to preclude homeologous pairing, as has been suggested for the natural allopolyploid Arabidopsis suecica [32] , or C. sativa similar to wheat and canola may have established the diploid behaviour of the sub-genomes through genetic control of aberrant pairing [32] . Polyploidization generally evokes a myriad of genetic and epigenetic responses resulting in expression variation and novel regulatory interactions, which is thought to lead to subfunctionalization or neofunctionalization of duplicated genes [29] , [33] , [34] . The genome Cs-G3 shows some evidence of expression dominance and a small proportion of the triplicated genes (22%) suggest functional diversification. However, the overall expression landscape of C. sativa supports preferential sheltering of duplicated genetic material, which would accommodate buffering of essential functions and maintenance of gene dosage balance. Polyploidy has commonly been associated with increased allelic diversity, heterozygosity and fixed heterosis, contributing to increased vigour, productivity and novel phenotypic variation, with the resultant prevalence of this phenomenon among crop species. The triplicated gene repertoire of C. sativa may be the genetic basis of several of its desirable agronomic and oil-quality attributes. One of the challenging practical consequences of the homogenous polyploid genetic code in C. sativa is that most traits will be controlled by multiple loci, where both traditional breeding and gene manipulation approaches will be more difficult. However, knowledge of the genome organization of C. sativa combined with ongoing efforts directed towards characterization of its transcriptome and germplasm diversity will accelerate future breeding of elite cultivars and designer oilseed lines for the biofuel and chemical industries. Plant material and nuclear DNA isolation A homozygous doubled haploid line DH55, derived from C. sativa genotype SRS 933, was chosen for sequencing. For nuclei isolation, ~40 g of fresh leaf tissue from 4-week-old etiolated DH55 seedlings was homogenized in 200 ml ice-cold homogenization buffer (0.01 M Trizma base, 0.08 M KCL, 0.01 M EDTA, 1 mM spermidine, 1 mM spermine, 0.5 M sucrose plus 0.15% β-mercaptoethanol, pH 9.4–9.5). The homogenate was filtered through two layers of cheesecloth and one layer of miracloth, and the nuclei pelleted by centrifugation at 1,800 g at 4 °C for 20 min. The pellet was resuspensed in wash buffer (1 × homogenization buffer plus 0.5% Triton-X100) followed by centrifugation at 1,800 g at 4 °C for 15 min, three times. After the final wash, the nuclei were resuspended in 10 ml lysis buffer (100 mM TrisCl, 100 mM NaCl, 50 mM EDTA, 2% SDS). High-molecular weight genomic DNA was then extracted by traditional proteinase K (0.05 mg ml −1 ; 65 °C for 2 h) digestion followed by RNAase A treatment, two cycles of phenol/chloroform extraction and ethanol precipitation. Quantification of genomic DNA was performed using PicoGreen dsDNA kit (Molecular Probes). Library construction and sequencing Genomic DNA (5–40 μg) was randomly sheared using the Covaris S2 ultrasonicator (Covaris Inc.), Hydroshear (Genomic Solutions Inc.) or gas-driven nebulizers. For Illumina sequencing, two paired-end (PE) libraries (with median insert sizes of 225 and 325 bps; Supplementary Table 1 ) and three short-span mate-paired (MP) libraries (3, 5 and 8 Kb) were constructed following standard TruSeq DNA sample preparation and MP library preparation kit v2 (Illumina), respectively. All libraries were size-selected using Pippin prep automated gel electrophoresis system (Sage Science), quantified using a Bioanalyzer (Agilent) and KAPA library quantification kit for Illumina (KAPA Biosystems) and sequenced from both ends (PE) for 100 cycles on an Illumina HiSeq 2000 instrument. For 454 pyrosequencing, three medium-span MP libraries with median insert sizes of 15, 20 and 25 kb ( Supplementary Table 1 ) were constructed following the method described in the GS FLX Titanium 20-kb span MP library preparation manual from Roche. Additionally, for 454 pyrosequencing, we constructed a long-span fosmid-based 40 kb MP library using NxSeq 40-kb MP cloning kit (Lucigen) with several modifications to the manufacturer’s protocol. A detailed protocol is described in Supplementary Note 6 . These libraries were sequenced using a Roche 454 FLX Titanium sequencer. Genome assembly Before assembly, all Illumina and 454 reads were filtered for adapter contamination, PCR duplicates, ambiguous residues (N’s) and low-quality regions, as described in Supplementary Note 7 . The initial backbone of the draft genome was assembled with Illumina reads using De Bruijn graph-based SOAPdenovo (version 2.01) assembler [35] , run with a kmer parameter of 47 (selected after testing a range of kmer values between 31 and 55) and each library ranked according to insert size from smallest to largest. The gaps within assembled scaffolds were filled with the short insert (225 and 325 bp) PE reads using GapCloser (version 1.12) [35] . The resulting assembly consisted of a total of 39,514 contigs and short scaffolds, with a sequence span of 641.39 Mb and an N50 size of 603 kb ( Supplementary Table 2 ). To improve the scaffold size, we used Bambus [36] to overlay the MP information generated by 454 pyrosequencing onto SOAPdenovo scaffolds. To achieve this, 454 MP reads of 15–40 kb span were aligned to SOAPdenovo scaffolds using a genomic mapping and alignment programme (GMAP) [37] . The output from GMAP was used to create a Bambus-compatible GDE-formatted contig file as a source of information about scaffold links. MP links were checked for validity. Redundant or multi-mapped mates were considered invalid; additionally, mates where only one read mapped or if both mates mapped to a single scaffold were also ignored. Thus, only MPs that uniquely mapped against two independent scaffolds with no overlap were considered valid. Bambus was run in a hierarchical fashion (each MP link considered in ascending order of their length) with scaffolding parameters, including redundancy (minimum number of links required to connect two scaffolds) level of 2 and link-size error (estimated error in mate span determination) of 5%. By default, the scaffolds resulting from Bambus are potentially ambiguous as two or more contigs may occupy the same place in the genome [36] . Such situations may occur either due to misassembled repeats, or when assembling homeologs within polyploid plant genomes. We used the ‘untangle’ utility of Bambus to disambiguate such scaffolds and generate a collection of linear scaffolds. Bambus was able to order, orient and merge 5,247 of these pre-assembled SOAPdenovo scaffolds into 3,206 superscaffolds, resulting in a greatly improved assembly with an N50 size of 2.16 Mb ( Supplementary Table 2 ). High-density genetic mapping and anchoring of the genome To order, orient and anchor Bambus scaffolds along the chromosome, a high-density genetic map representing 20 linkage groups was constructed using a mapping population (F6) of 96 recombinant inbred lines derived previously from a cross between the phenotypically distinct C. sativa cultivars Lindo and Licalla [1] . A total of 3,575 polymorphic loci (SNPs, simple sequence repeats and insertion/deletion polymorphisms; Supplementary Table 3 ), identified by a combination of the GoldenGate genotyping assay (Illumina) and RAD (Restriction site Associated DNA) [38] approaches, were used to integrate Bambus superscaffolds with the genetic map. To further assist with ordering and orientation of scaffolds for which there was paucity of adequate genetic recombination and markers, collinearity between C. sativa provisional pseudomolecules and A. thaliana chromosomes or A. lyrata scaffolds was established using NUCmer [39] and BLASTP [40] . A total of 57 instances of false joins or insertions within Bambus superscaffolds were identified based on marker discontiguity and collinearity information. Such misassembled scaffolds were split and the correct position of each of the fragments was determined based on marker and collinearity information. Final scaffolds were renamed as ‘Scaffold’ and numbered sequentially based on their length from longest to shortest. The order and orientation of scaffolds within each pseudomolecule was determined based on marker order within each scaffold, and marker contiguity pattern between adjoining scaffolds. Scaffolds with too few markers were ordered and oriented using collinearity information. The final version of the draft genome representing 20 pseudochromosomes (corresponding to 20 linkage groups) and 37,398 unanchored scaffolds was collated using a custom Perl script, and the ordering and orientation information of scaffolds within each pseudochromosome was compiled in AGP files. The quality of the assembled genome was ascertained by performing several independent tests, as described in Supplementary Note 3 . Repeat annotation Using the assembled C. sativa genome as input, a de novo repeat library was constructed by using RECON and RepeatScout within RepeatModeler (Version 1.05; http://www.repeatmasker.org/RepeatModeler.html ). To reduce potential false positives, repetitive sequences were compared (BLASTX with E-value cutoff of 1E−5) with annotated gene models in the A. thaliana protein database and significant non-TE hits were removed. The final consensus repeat library was used to mask the genome by RepeatMasker (Version 3.3.0; http://www.repeatmasker.org/RMDownload.html ). Gene annotation For accurate annotation of gene models, an integrated computational approach ( Supplementary Fig. 4 ) based on two major annotation pipelines, Maker [41] and PASA [42] , was adopted. Maker provides a simplified process for aligning ESTs and proteins to the genome, and integrates this external homology evidence with ab initio gene predictions to produce final gene annotations with evidence-based quality statistics. Inputs for Maker included the repeat-masked C. sativa genome assembly, 42,350 ESTs, a genome-guided de novo transcript assembly comprising 201,365 transcripts and a protein database containing annotated proteins from A. thaliana , A. lyrata , B. rapa and Thellungiella parvula . Ab initio gene predictions were made by Fgenesh [43] and Augustus [44] . Maker gene structure annotations were further updated by PASA using evidence from de novo RNA-seq assembly and Sanger/454 ESTs. Annotation updates by PASA included annotation of untranslated regions, addition of models for alternative splicing variants and gene boundary adjustments. A total of 84,071 genes were annotated by this approach, of which 7,175 genes were identified as ‘fused’ where two or more neighbouring A. thaliana genes aligned (BLASTN with E-value cutoff of 1E−10) to different parts of a single predicted gene model in C. sativa . The fused genes were replaced with 12,984 alternative gene models and the output was passed through another round of PASA. By manual curation, 793 EST-only or other predictions that overlapped with gene models that had better external homology evidence support were removed. The final annotation set contained a total of 89,418 genes encoding 94,495 transcripts. Synteny analysis Sequence homology was detected by BLASTP of the predicted proteins against A. thaliana proteome. BLAST hits with E-value of 1e−20 or better and within the top 40% drop from the best bit score were kept for further analysis. The chains of syntenic C. sativa – A. thaliana gene pairs were computed by DAGChainer [45] using default parameters. In case of a C. sativa gene participating in more than one syntenic chain due to duplication in the A. thaliana genome, the C. sativa – A. thaliana pair in the weaker scoring chain was removed from the analysis. The syntelog table was generated by placing the syntenic chains onto the C. sativa chromosomes. Reconstruction of triplicated sub-genomes within C. sativa Considering the high level of conservation of synteny and GB contiguity between C. sativa and Arabidopsis species, the A. lyrata genome was utilized to represent the genome organization of individual sub-genomes within C. sativa . Since the prevalence of inversions and intrachromosomal rearrangements is thought to be more common than interchromosomal translocations [23] , segments of each C. sativa chromosome syntenic to corresponding A. lyrata chromosomes were assumed to be derived from the same ancestral chromosome. In the event where interchromosomal rearrangements were inferred, the order, orientation and contiguity of genes across potential adjacent segments were examined, and the most parsimonious scenario for the original segment order and chromosome assignment within each sub-genome was deduced. Transcriptome sequencing The whole-plant transcriptome of C. sativa based on Illumina RNA-seq data was characterized to assist in the genome annotation process. Twelve different tissue samples were collected during both vegetative (germinating seed, cotyledon, young leaf, senescing leaf, root and stem) and reproductive (bud, flower, and early, early-mid, late-mid and late seed development) stages of the life cycle ( Supplementary Table 10 ). For each tissue type, at least three independent biological replicates were analysed. Total RNA from vegetative tissue was isolated using the RNeasy plant mini kit (Qiagen), including on-column DNase digestion, according to the manufacturer’s instructions. Total RNA from siliques was isolated using a method described by Suzuki et al. [46] , consisting of a two-step extraction process with high sodium extraction buffer isopropanol precipitation and LiCl precipitation, and then cleaned using RNeasy plant Mini kit (Qiagen), including on-column DNase digestion. The integrity and quantity of total RNA was assessed using RNA 6000 Nano labchip on the BioAnalyzer (Agilent). Sequencing libraries were constructed following standard TruSeq RNA sample preparation guide (Illumina) and multiplexed (12 samples per lane of a flow cell), PE sequencing was performed using the Illumina Hiseq 2000 platform. A total of 78.5 Gb raw RNA-seq data was generated. Before assembly, all reads were filtered for adapter contamination, ambiguous residues (N’s) and low quality regions, as described in Supplementary Note 7 . De novo assembly of transcripts and expression analysis was performed using a combination of different programs, including Tophat [47] , Cufflinks [47] , Trinity [48] and PASA [42] . Clean and non-ribosomal reads from one biological replicate of each tissue sample were pooled and used for genome-guided de novo transcript assembly. A hybrid approach combining three different programs, including Tophat, Trinity and PASA, was employed to align RNA-seq reads to the genome (Tophat), assemble aligned reads (Trinity) and further align and assemble the Trinity-reconstructed transcripts (PASA). This approach produced 201,365 transcripts, which were used in the annotation of protein-coding genes in the C. sativa genome ( Supplementary Fig. 4 ). For de novo transcriptome assembly, clean and non-ribosomal reads from all tissue samples (including all three biological replicates) were pooled. De novo assembly was carried out using Trinity with default parameters. The final assembly included 271,745 Trinity transcripts and 115,114 Trinity components, which were used for updating Maker gene structure annotation using PASA ( Supplementary Fig. 4 ). To estimate transcript abundance, the whole-plant and tissue-wise expression of C. sativa genes was assessed using a Tophat and Cufflink-based method [47] . For both Tophat and Cufflink analysis, default parameters were used except that the maximum and minimum intron lengths were set at 2,500 and 20, respectively. For whole-plant-wide expression analysis of C. sativa genes, RNA-seq data from all tissues and biological replicates were pooled. Transcript abundance was measured as fragments per kilobase of exon per million fragments mapped (FPKM) values. For all the 18,565 fully retained Camelina sativa genes, the raw expression values (FPKM) from each of the 12 tissue types were transformed by adding 1 and taking the natural logarithm, in order to analyse expression divergence. All subsequent calculations were done with the transformed values. This transformation reduces the range of the data, and the residuals more frequently follow a normal distribution (determined by the distribution of P values for the Shapiro–Wilk test for normality), which is an assumption of ANOVA. Of the gene triplets, 18,491 had non-zero variance of expression. For the expression analyses, the mean was taken over the three replicates, for each sub-genome of origin (G) and tissue type (T) combination. The mean for each G was also obtained (over all T and replicates). Two-way ANOVAs were carried out to test for the interaction between the G effect and the T effect on expression in addition to the sum of these separate effects. The cumulative frequency of each genome demonstrating the highest expression ( Fig. 6b ) was obtained after sorting the gene triplets into increasing order of P value (ANOVA test for interaction, based on a sample size of 108 per gene triplet (3 genes by 12 tissue types by 3 replicates)) for the G × T effect. Of the 18,491 gene triplets, 14,391 showed a significant ( P <0.05; ANOVA test for interaction) G × T interaction effect. However, in most cases due to small statistical error the interaction was small in magnitude despite its statistical significance. The magnitude of interaction σ i was estimated as the square root of the variance of the interaction in the random effects model [49] that considers the levels of G and T as randomly sampled. This estimate was obtained from equation (1) where E stands for expectation, and the expected MS terms are the expected mean squares calculated as in ANOVA, and n is the number of replicates (in this case 3). The scatterplot ( Fig. 6c ) illustrates the relationship between these two measures of the interaction. Only 4,106 triplets are both statistically significant ( P <0.05; ANOVA test for interaction) and have a magnitude of interaction σ i >0.25. From this set, only the individual genes (12,112) that had a non-zero expression for at least one tissue type were considered for hierarchical clustering. The clustering was carried out using 1 minus the Pearson sample correlation as the distance measure, and this requires the sample variances of the means for each gene to be non-zero. These sample variances were only zero in the case that all the means were zero. The average linkage method was used for clustering. This method clusters correlated sets of expression means together regardless of the absolute magnitude of the expression levels. Using this clustering, the heatmap ( Supplementary Fig. 12 ) was drawn using the statistical package R where the colours were 256 levels of rainbow, starting with red representing low values and ending with blue representing high values. The superimposed pink-coloured rectangles highlight areas of low or high expression. The breakpoints determining the y coordinates of the rectangles were also chosen with reference to the dendrogram for the clustering such that they separated clearly defined clusters of genes having similar expression patterns. Identification of orphan genes A blast-based filtering approach was used to identify orphan genes in the C. sativa genome. BLASTP (E-value cutoff of 0.01) was used to search all predicted peptides of C. sativa against all 39 sequenced plant species available at phytozome.net (v9.1) excluding five Brassicaceae species. The orphan candidates were filtered out, and then BLAST searched against the NCBI nr, nt and est databases (E-value cutoff of 0.01). Orphans having significant blast hits with Brassicaceae species were filtered out. The species and family information of all the candidates were extracted from the NCBI taxonomy database using in-house developed scripts. Filtered candidates were further searched against the nr database using PSI-BLAST. Orphan candidates displaying InterProScan hits with non-Brassicaceae species were not considered as orphans. C. sativa specific orphans were extracted from the 3,761 Brassicaceae-specific orphans by BLAST search of these genes against the C. sativa genome. Identification of evolutionary origins of orphan genes C. sativa orphan genes originating by gene duplication events were identified by BLASTP and BLASTN searches against all non-orphan C. sativa genes. Orphan genes containing non-coding or out-of-frame CDS hits were identified using BLASTN against all sequenced plant species, and hits with Brassicaceae and non-Brassicaceae species were categorized. An orphan gene was considered to be overprinted if the peptide sequence of orphan overlapped with the CDSs of other genes (not with untranslated regions or intronic regions). BAC library construction and sequencing A ~10-fold coverage BAC library of C. sativa was constructed in the pIndiogoBAC vector by Bio S&T Inc. (Montreal, Canada). Young etiolated leaves from seedlings of DH55 were used as source material for BAC library construction. A subset of 768 randomly selected BACs was sequenced by Amplicon Express Inc. (Pullman, WA, USA) by Focused Genome Sequencing, a next-generation sequencing-based method that allows high-quality assembly of BAC clone sequence data using the Illumina platform. Phylogenetic analysis of Camelina species De novo transcriptome sequencing of five Camelina species, including C. hispida, C. rumelica ssp. transcaspica, C. rumelica ssp. Iran, C. rumelica ssp. USSR and C. laxa , was performed using Roche 454 pyrosequencing ( Supplementary Table 22 ). The unigene sets generated by de novo EST assembly were utilized in establishing a highly resolved molecular phylogeny of Camelina species and their relationship with the three sub-genomes of C. sativa . Additional information is provided in Supplementary Note 5 . Accession codes: Sequence data for Camelina sativa have been deposited in DDBJ/EMBL/GenBank sequence read archive under the accession codes SRP038024 , SRS558774 , SRS566487 and SRS559344 . The genome assembly for Camelina sativa has been deposited in DDBJ/EMBL/GenBank nucleotide core database under the accession code JFZQ00000000 . How to cite this article: Kagale, S. et al. The emerging biofuel crop Camelina sativa retains a highly undifferentiated hexaploid genome structure. Nat. Commun. 5:3706 doi: 10.1038/ncomms4706 (2014).